Magnetic spin imaging under ambient conditions with sub-cellular resolution The detection of small numbers of magnetic spins is a significant challenge in the life, physical and chemical sciences, especially when room temperature operation is required. Here we show that a proximal nitrogen-vacancy spin ensemble serves as a high precision sensing and imaging array. Monitoring its longitudinal relaxation enables sensing of freely diffusing, unperturbed magnetic ions and molecules in a microfluidic device without applying external magnetic fields. Multiplexed charge-coupled device acquisition and an optimized detection scheme permits direct spin noise imaging of magnetically labelled cellular structures under ambient conditions. Within 20 s we achieve spatial resolutions below 500 nm and experimental sensitivities down to 1,000 statistically polarized spins, of which only 32 ions contribute to a net magnetization. The results mark a major step towards versatile sub-cellular magnetic imaging and real-time spin sensing under physiological conditions providing a minimally invasive tool to monitor ion channels or haemoglobin trafficking inside live cells. Improvements to current magnetic resonance imaging (MRI) techniques will allow chemical analysis of samples with high resolution down to sub-cellular volumes. However, conventional magnetic imaging is hindered by inductive detection requiring a sufficient magnetic flux from the sample to induce a detectable current in the pickup coil. Increases in spatial resolution reduce the number, n, of detected spins until the statistical polarization, whose magnitude is of order [1] , exceeds the magnetization due to Boltzmann polarization. The resultant vanishing mean field strength and its stochastic nature render common detection schemes ineffective. Precision magnetometers provide exceptional sensitivities reaching a few fT/√Hz [2] , [3] , [4] , [5] , yet their relatively large size and/or operational conditions prohibit sensing of small numbers of spin magnetic moments at ambient conditions and sub-micron resolution. Sensors based on nitrogen-vacancy (NV) centres in diamond are promising magnetometers because of their atomic size. This allows placement of the sensor with few nanometre proximity to the sample while retaining superior volume-to-sensitivity scaling, room temperature operation and optical readout [6] , [7] , [8] . Precision metrology has already been demonstrated for DC and AC fields [9] , [10] , [11] , [12] , [13] , [14] , spins within the diamond lattice [15] , [16] , [17] , [18] and surface spins [19] . Here, we demonstrate sensing and imaging of stochastic magnetic fluctuations originating from freely diffusing electron spins such as paramagnetic oxygen (O 2 , S =1), MnCl 2 ( S =5/2) and Gadolinium ions (Gd 3+ , S =7/2) in liquids, immobilized in polymers and linked specifically to cellular structures. NV relaxometry In low external magnetic fields, freely diffusing ions exhibit a zero-mean field, but magnetic field fluctuations due to statistical spin polarization cause a non-zero RMS field with random phase. Such stochastic fields are difficult to detect, but the NV offers a striking avenue to measuring such random fields by monitoring its quantum relaxation [20] , [21] . To benefit from ensemble sensing sensitivity [22] , [23] , we employ an array of atomic sized NV sensors (~1,000 μm − 2 ) with a calculated mean depth of h =6.7 nm (ref. 24 ), as illustrated in Fig. 1 . After preparation of a distinct NV spin state, interaction with the environment leads to NV relaxation with rate Γ=Γ int +Γ env . The contributions intrinsic to the diamond, Γ int , include spin impurities and vibrational lattice dynamics, whereas Γ env depends on the external environment to which the system can deliberately be exposed. Relaxation may occur via the transverse and longitudinal relaxation channels characterized by their respective decay times T 2 and T 1 . The transverse dephasing rate Γ 2 =1/ T 2 is increased by fluctuations at low frequencies (kHz to MHz) and can be monitored using spin echoes or higher order dynamical decoupling microwave control protocols [25] , [26] , [27] . The longitudinal relaxation rate Γ 1 =1/ T 1 describes the population decay of a polarized spin into thermal equilibrium. It is susceptible to frequencies at the NV Larmor precession ω 0 = D ± γB 0 , where γ is the gyromagnetic ratio and B 0 is a magnetic offset field. Owing to the large NV zero-field splitting of D =2.87 GHz this is in the GHz range at low fields. 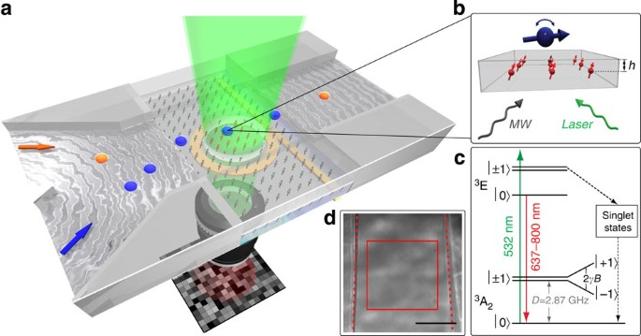Figure 1: Widefield magnetometry with microfluidic detection. (a,b) Widefield excitation (green) of the NV spin array (red arrows) and spatially resolved CCD detection of NV fluorescence. Homogeneous spin manipulation of the NV array is achieved via a lithographic Ω-microwave structure (yellow). Gd3+ions (blue spheres ina,bin aqueous solution are introduced using a microfluidic channel placed directly on top of the sensor proximal to the NV array withh=6.7 nm. (c) Energy level scheme of NV centre illustrating the high fluorescent signal extending from 637–800 nm. The |0› spin sublevel has a stronger fluorescence than the |±1› states as they emit less photons owing to a higher probability to enter the long-living singlet states. NV relaxation is thus readout optically. (d) Brightfield image of the microfluidic channel with channel boundaries (dotted lines) and 30 × 30 μm2detection region of interest (ROI, red rectangle). Scale bar, 20 μm. Figure 1: Widefield magnetometry with microfluidic detection. ( a , b ) Widefield excitation (green) of the NV spin array (red arrows) and spatially resolved CCD detection of NV fluorescence. Homogeneous spin manipulation of the NV array is achieved via a lithographic Ω-microwave structure (yellow). Gd 3+ ions (blue spheres in a , b in aqueous solution are introduced using a microfluidic channel placed directly on top of the sensor proximal to the NV array with h =6.7 nm. ( c ) Energy level scheme of NV centre illustrating the high fluorescent signal extending from 637–800 nm. The |0› spin sublevel has a stronger fluorescence than the |±1› states as they emit less photons owing to a higher probability to enter the long-living singlet states. NV relaxation is thus readout optically. ( d ) Brightfield image of the microfluidic channel with channel boundaries (dotted lines) and 30 × 30 μm 2 detection region of interest (ROI, red rectangle). Scale bar, 20 μm. Full size image Spin noise sensing First, we demonstrate magnetic sensing of various chemical environments by probing both relaxation channels along one preferred NV axis ( B 0 =5 mT) in the presence of air, water and a solution of 1 M Gd 3+ (see Table 1 ). Particularly the large magnetic moment of Gd 3+ has made the Gd 3+ chelate a prime candidate as relaxation contrast agent in MRI [28] . In this system, probing Γ 2 by a Hahn echo sequence shows only marginal changes in T 2 for Gd 3+ , while multi-pulse CPMG81 is mildly responsive with a change in T 2 of 13.5%. The longitudinal T 1 , however, exhibits a prominent reduction of 94% in the presence of Gd 3+ and was similarly responsive to dissolved MnCl 2 and with O 2 saturated water ( Fig. 2a and Supplementary Fig. S1 ). Focusing on the dominant Gd 3+ , the relaxation rate Γ Gd induced by freely diffusing Gd 3+ depends on the corresponding RMS magnetic field and its spectral density S Gd ( ω ). For a Gaussian process, the latter is given by , where ω 0 is the Larmor frequency of Gd 3+ . Boltzmann polarization and ω 0 can be neglected for the low B 0 fields applied. S Gd ( ω ) is instead dominated by statistical polarization and substantial broadening effects of zero-mean fluctuations f Gd = f dipole + f vib + f trans + f rot . The contribution from the concentration-dependent dipole coupling between the Gd 3+ is given by f dipole = c Gd ·77 GHz M −1 ( Supplementary Note 1 ), where c Gd is the spin concentration in mol l −1 . Intrinsic vibrational spin relaxation of the complexed Gd 3+ ion yields a constant fluctuation of f vib ~50 GHz [29] , while rotational motion f rot and translational diffusion f trans cause fluctuations of ~140 MHz ( Supplementary Fig. S2 ). The resulting broadening of the spectral density S Gd ( ω ) is therefore effectively constant up to a few tens of GHz ( Fig. 2b ), where resonant Gd 3+ -induced fluctuations B x and B y (NV axis defines z) cause Γ 1 relaxation of the NV. The magnetic field variance is derived from the dipolar NV-Gd 3+ coupling and is given by Table 1 Transverse ( T 2 ) and longitudinal ( T 1 ) NV spin relaxation in various environments. 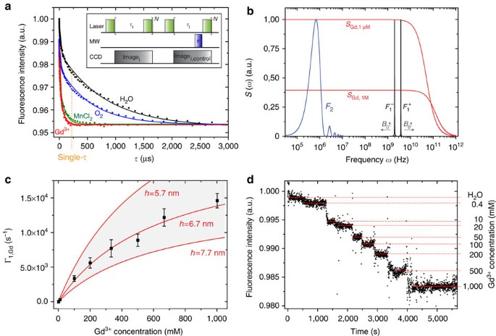Figure 2: Microfluidic spin sensing. (a)T1relaxation curves of the NV ensemble in the presence of water (black), oxygenated water (~1.5 mM, blue), 1 M MnCl2(green) and 1 M Gd3+(red). Solid curves are bi-exponential fits to the data. Optimized spin detection via direct fluorescent readout is achieved at a discrete interrogation period τ (orange). The inset shows the measurement pulse sequence and normalization. (b) Spectral densitySGd(ω)of Gd3+for two distinct concentrations (red curves) illustrating the broadening effect due to Gd3+coupling (fdipole) at higher concentrations. Although the sensitivity windows ofT2-decoherence (F2, blue) is limited to low MHz fluctuations,T1-relaxometry allows to probe a wide frequency range up to GHz with two sensitivity windows (F1−andF1+, black).can be Zeeman-shifted viaB0enabling experimental detection ofSGd(ω). (c) Experimental relaxation rate Γ1,Gdas a function of the Gd3+concentration (black squares with 1 σ s.e. and three independent measurements) and analytical predictions for specific mean implantation depthsh(red curves). (d) Dynamic microfluidic single-τ detection (τ=100 μs) of varying Gd3+concentrations with a single data point acquisition time oftm~2 s. Full size table Figure 2: Microfluidic spin sensing. ( a ) T 1 relaxation curves of the NV ensemble in the presence of water (black), oxygenated water (~1.5 mM, blue), 1 M MnCl 2 (green) and 1 M Gd 3+ (red). Solid curves are bi-exponential fits to the data. Optimized spin detection via direct fluorescent readout is achieved at a discrete interrogation period τ (orange). The inset shows the measurement pulse sequence and normalization. ( b ) Spectral density S Gd (ω) of Gd 3+ for two distinct concentrations (red curves) illustrating the broadening effect due to Gd 3+ coupling ( f dipole ) at higher concentrations. Although the sensitivity windows of T 2 -decoherence ( F 2 , blue) is limited to low MHz fluctuations, T 1 -relaxometry allows to probe a wide frequency range up to GHz with two sensitivity windows ( F 1 − and F 1 + , black). can be Zeeman-shifted via B 0 enabling experimental detection of S Gd (ω) . ( c ) Experimental relaxation rate Γ 1,Gd as a function of the Gd 3+ concentration (black squares with 1 σ s.e. and three independent measurements) and analytical predictions for specific mean implantation depths h (red curves). ( d ) Dynamic microfluidic single-τ detection (τ=100 μs) of varying Gd 3+ concentrations with a single data point acquisition time of t m ~2 s. Full size image where N A is the Avogadro constant, μ 0 the vacuum permeability, h the mean depth of the NV centres and γ NV ≈ γ Gd ( Supplementary Fig. S4 ). The effective RMS field strength is then given by . The time-dependent probability of finding the NV in the |0› state ( Supplementary Note 2 ) is given by where are the individual decay rates of each sensitivity window ( Fig. 2b ) integrated over S Gd ( ω ). The overall decay rate Γ 1,Gd of the longitudinal NV magnetization is then given by This theoretical prediction was experimentally verified by varying c Gd ( Fig. 2c ), showing excellent agreement for the non-trivial dependence on c Gd . At nanometre length scales, the sample-sensor distance is a key parameter as and thus represents a viable tool to access the average implantation depth of nitrogen ions ( Fig. 2c ). The relaxometric SNR=Γ Gd /Γ int of T 1 is much higher as Γ 2,int »Γ 1,int due to the low spin-orbit coupling accompanied by a low phonon density in diamond [30] . Hence, in this system longitudinal T 1 outperforms T 2 -relaxometry by two orders of magnitude ( Supplementary Fig. S3 ) and is employed from here on. Microfluidic single-τ detection Next, we optimized the microfluidic detection by converting the T 1 signal directly into a measureable fluorescence. Instead of detecting the full relaxation curve, the fluorescent NV response at a single-τ point is utilized as direct concentration readout ( Fig. 2a ). Maximum sensitivity is achieved at τ~ T 1,Gd /2 for c Gd <10 mM and approaches T 1,Gd for higher c Gd ( Supplementary Note 4 and Supplementary Figs S6–S8 ). Therefore, varying Gd 3+ concentrations can be monitored dynamically with temporal resolutions in the order of a second ( Fig. 2d ). For maximal sensitivity all four crystallographic NV orientations can be employed, as exhibits a random magnetic field orientation. This is achieved by measuring in near-zero field (50 μT earth field) and probing all NV orientations at D =2.87 GHz, which effectively improves the fluorescent single-τ contrast and increases the number of sensing NV spins by a factor of four ( Supplementary Fig. S9 ). We applied a statistical t -test (2 σ) to the fluorescence traces to identify the lowest concentration still significantly different to pure water. After a total measurement time of t m =20 s and an optimized τ=400 μs, we resolved =250 μM and 80 μM for single and all four NV axes, respectively. In addition, the multiplexed charge-coupled device (CCD) detection allows varying the detection voxel equivalent to an effective change in spatial resolution of magnetic sensing. For fixed t m and CCD detection, depends on the shot noise of detected photons and thus on the applied pixel binning ( Supplementary Fig. S3 ). Although single pixel analysis is feasible, the lower limit of the spatial resolution for the widefield detection is Δ r xy ~430 nm ( Supplementary Fig. S10 ). In our experimental setup this translates into 4 × 4 pixels (equivalent to Δ r xy ~460 nm). For such a small voxel, we detected =500 μM, which approaches typical ion concentrations encountered in oxidative bursts [31] or senile placques [32] . As demonstrated previously, lower spin concentrations can conveniently be sensed by spatially averaging over larger voxels. To determine the sensitivity in terms of number of spins per detection voxel we emphasize that Γ 1,Gd integrates the signal from the spins above the surface while proximal ions ( r = h ) contribute most due to the h −3 scaling. We determined the height dependence by employing polymer spacers between NV and Gd 3+ , which yielded a decay of Γ 1,Gd ( r ) to 1/e at Δ r z =15 nm ( Supplementary Fig. S11 ). Taking the experimental sensitivity to =500 μM detected in t m =20 s and a spatial resolution of Δ r xy =460 nm (4 × 4 pixels), this corresponds to an experimental detection of 1,000 statistically polarized spins of which only 32 ions contribute to an effective net magnetization. This spin sensitivity is an improvement by more than four orders of magnitude compared with other state-of-the-art magnetic sensing techniques operating at ambient conditions [33] , [34] , [35] . Single spin detection has been demonstrated using magnetic resonance force microscopy [3] , [8] , but at the expense of cryogenic temperatures and significantly longer acquisition times. The combination of spatio-temporal resolution, spin sensitivity and the operability under ambient conditions using widefield NV relaxometry paves the way towards minimally invasive real-time observation of chemical and biological processes involving magnetic spins on the sub-cellular level. Relaxometric imaging Finally, this unprecedented spatial-temporal resolution is used to image magnetic fluctuations originating from samples on the sensor array ( Fig. 3a ). A periodic grid of lithographically patterned Gd 3+ is easily resolvable in the reconstructed T 1 image ( Fig. 3b ). However, t m can be reduced by orders of magnitude applying the optimized single-τ detection, yielding yet higher contrast of magnetic imaging ( Fig. 3c ). For high-resolution magnetic imaging in biological samples, we have specifically labelled the plasma membrane of HeLa cells with caged Gd 3+ ions and an Alexa532 fluorophore via biotinylated poly- L -lysine. As the NV sensor is most sensitive to proximal spins, we placed 150 nm thin ultramicrotome sections of labelled cells onto the diamond sensor. The control fluorophore indicates a successful label of the magnetic marker to HeLa cells ( Fig. 3d ), while the boundary of the cell is clearly present in the magnetic image ( Fig. 3e ). Furthermore, a line scan through the magnetically labelled plasma membrane verifies a spatial resolution of Δ r xy =472 nm approaching the inherent optical limit of the conventional widefield technique. A complete simulation of the single-τ detection based on shot noise limited photon detection agrees with the experimental sensitivities ( Fig. 4 , Supplementary Fig. S8 ). The key advantage of magnetic spin labels is the potential for chemically selective spin contrast imaging as each spin label is expected to have a distinct S(ω) , for example, by binding to a certain biological complex. Using the NV, the spectral density can be measured with a high bandwidth as Γ 1 provides a narrow and via B 0 tunable sensitivity window (F 1 in Fig. 2b , experimental realization in Supplementary Note 3 and Supplementary Fig. S5 ). 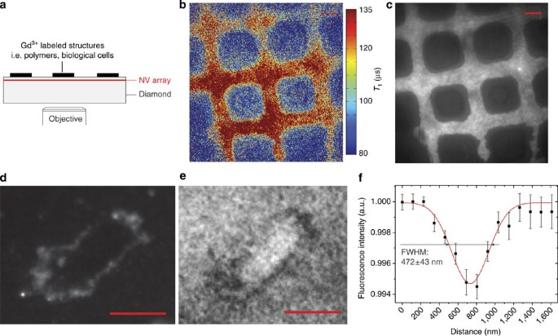Figure 3: Spin contrast imaging. (a) Schematic of magnetic spin imaging. (b)T1weighted image of lithographically patterned Gd3+grid (blue rectangular regions with lowT1) on top of diamond sensor. Three data sets, each containing the fullT1-decay information with varying τ, were acquired withintm=45 min, subsequently averaged and fitted to obtainT1for each pixel. (c) Single-τ imaging (τ=150 μs) directly yields dark areas where Gd3+is present due to the increased NV relaxation. Although a single image (tm=2 s) is sufficient to identify the pattern, the image shown was averaged for 10 min to enhance the contrast. (d) Fluorescent control image of an ultramicrotome sectioned HeLa cell (150 nm), where the plasma membrane was labelled with biotin-poly-L-lysine-Gd3+-DTPA-Alexa532 (Alexa532 fluorescence spectrally filtered from 550–575 nm). (e) Magnetic imaging via a single-τ measurement (tm=15 min, τ=440 μs,B0~50 μT) evidencing the presence of magnetic Gd3+at the cell membrane (dark structures). (f) Line scan through plasma membrane shown in (e) demonstrating spatial resolution of 472 nm. Errors bars, 1 σ s.e. of six independent line scans. Scale bars, 5 μm. Figure 3: Spin contrast imaging. ( a ) Schematic of magnetic spin imaging. ( b ) T 1 weighted image of lithographically patterned Gd 3+ grid (blue rectangular regions with low T 1 ) on top of diamond sensor. Three data sets, each containing the full T 1 -decay information with varying τ, were acquired within t m =45 min, subsequently averaged and fitted to obtain T 1 for each pixel. ( c ) Single-τ imaging (τ=150 μs) directly yields dark areas where Gd 3+ is present due to the increased NV relaxation. Although a single image ( t m =2 s) is sufficient to identify the pattern, the image shown was averaged for 10 min to enhance the contrast. ( d ) Fluorescent control image of an ultramicrotome sectioned HeLa cell (150 nm), where the plasma membrane was labelled with biotin-poly- L -lysine-Gd 3+ -DTPA-Alexa532 (Alexa532 fluorescence spectrally filtered from 550–575 nm). ( e ) Magnetic imaging via a single-τ measurement ( t m =15 min, τ=440 μs, B 0 ~50 μT) evidencing the presence of magnetic Gd 3+ at the cell membrane (dark structures). ( f ) Line scan through plasma membrane shown in ( e ) demonstrating spatial resolution of 472 nm. Errors bars, 1 σ s.e. of six independent line scans. Scale bars, 5 μm. 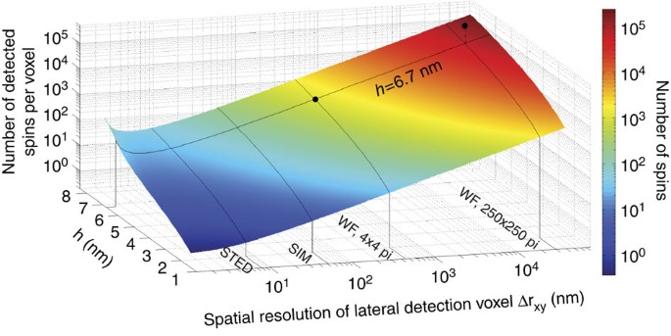Figure 4: Sensitivities of optimized single-τ detection. The minimum number of detectable spinsnGdwas simulated fortm=20 s as a function of sample-sensor distancehand spatial resolution Δrxy. Experimental results withh=6.7 nm and two distinct pixel binnings (black dots, WF: widefield detection) demonstrate good agreement. Fewer spins per voxel can be detected by decreasinghand/or the detection voxel equivalent to an increase in spatial resolution. Note thatT1,intremains to be experimentally determined for shallow NV depths withh<5 nm and is assumed to be constant for the simulation. Full size image Figure 4: Sensitivities of optimized single-τ detection. The minimum number of detectable spins n Gd was simulated for t m =20 s as a function of sample-sensor distance h and spatial resolution Δ r xy . Experimental results with h =6.7 nm and two distinct pixel binnings (black dots, WF: widefield detection) demonstrate good agreement. Fewer spins per voxel can be detected by decreasing h and/or the detection voxel equivalent to an increase in spatial resolution. Note that T 1,int remains to be experimentally determined for shallow NV depths with h <5 nm and is assumed to be constant for the simulation. Full size image The results presented here demonstrate highly sensitive minimally invasive spin sensing and imaging of unperturbed electron spins at room temperature. We have shown the NV-based relaxometric technique offers several advantages over other techniques capable of sensing statistical polarization [3] , [33] , [35] , [36] as it is operable under ambient conditions with no requirements of strong magnetic fields or radiofrequency pulses. Quantum relaxation of the NV sensor has the potential to emerge as a novel technique of high-throughput analytical sciences and contrast-enhanced optical-MRI at the nanoscale. A considerable improvement in sensitivity is possible by decreasing the NV depth h and the voxel size Δ r xy equivalent to enhancing the spatial resolution ( Fig. 4 and Supplementary Fig. S8 ). With h =2.5 nm and typical resolutions of Δ r xy =50 nm for structured widefield illumination [37] , a sensitivity in the order of ten Gd 3+ spins is expected. At the expense of longer integration, scanning techniques such as stimulated emission depletion would boost Δ r xy down to 8 nm [38] reaching even single spin sensitivities. Alternatively to our ensemble sensor, local spin densities could be monitored even inside living cells by employing single NVs embedded in nanodiamonds [39] , [40] . The high temporal resolution of widefield magnetometry favors sub-cellular visualization also of label-free dynamic processes, for instance the production of free radicals in cell death, the regulation of homoeostasis through ion channels [41] or haemoglobin trafficking by imaging paramagnetic oxygen. Experimental setup 15 N 2 at a fluence of 10 13 cm −2 with an energy of 4 keV per atom was homogeneously implanted into a 80-μm thin ultrapure type-IIa diamond (Element6) yielding a density of sensing NV spins of ~1,000 μm − 2 . According to a SRIM simulation (stopping and range of ions in matter) [24] , the mean depth of the NV sensor is h =6.7±2.8 nm. A 500 MHz PulseBlaster card (ESR-Pro-II, Spincore) was employed for timing the triggering of microwave pulses, CCD integration and the laser excitation. Laser (1.5 W of a 532- nm cw; Verdi, Coherent) was directed through an AOM (Crystal Technology) and focused onto the back-focal plane of a 60 × oil objective, 1.49 NA (Olympus). An 800 ns laser pulse allows optimal NV readout with subsequent re-polarization into the |0› ground state enabling CCD integration over multiple repetitions ( N ~10 4 per image). The fluorescent NV response was spectrally filtered (LP650, Omega) and projected onto a 512 × 512 cooled EM-CCD (CascadeII, Roper Scientific) yielding an effective pixel size of 115 nm. Homogeneous and resonant microwave manipulation of the NV sensor with an optical field of view of ~60 × 60 μm 2 was achieved using a lithographically grown broadband Ω-shaped structure. The flow rate in the microfluidic channel made of transparent polydimethylsiloxan (PDMS, Sylgard) was adjusted to 1 μl s −1 . All experiments were conducted with commercially available Gd 3+ solution (Gadovist, Bayer Schering Pharma), except for the spin contrast imaging of cellular structures (see cell preparation and synthesis of magnetic/fluorescent spin label in detailed method section). Alexa532 was imaged using a separate fluorescence filter (Semrock, HC 565/24). Cell culture, labelling and preparation In all, 2.5 × 10 6 HeLa ATCC cells were harvested and suspended in PBS buffer at a concentration of 25 × 10 6 cells per ml. Ten microlitre containing 20 mM solution of EZ-Link NHS Biotin (Pierce, 20217) in dimethylsulphoxide were added for 20 min to the cells for biotinylation. The cells were then fixed with 4% paraformaldehyde, extensively washed and resuspended in PBS buffer. After 5 min incubation with 100 μg streptavidin, cells were washed in PBS buffer, resuspended and incubated for 5 min with ~1 nmol of biotin-poly- L -lysine Gd-DTPA (see synthesis below). After extensive washing with PBS Puffer, cells were resuspended in 1 ml of 1.25 M sucrose solution and harvested by centrifugation. The cell pellets were mounted on an aluminium stub and vitrified by submersion in liquid nitrogen. Then, thin cell sections with a thickness of ~150 nm were produced with an Ultramicrotome (Leica UCT) equipped with a LKB Cryokit and freshly prepared glass knives (Leica KMR2). Frozen cell cuts were transferred onto the diamond under ambient conditions and embedded in PDMS to minimize changes in the refractive index. Synthesis of Biotin-poly- L -lysine-Gd 3+ -DTPA-Alexa532 Twenty-five microgram poly- L -lysine (Sigma-Aldrich, P2636) was dissolved in 0.1 M sodium hydrogencarbonate buffer (pH8.3). Then, 600 μmol diethylenetriaminepentaacetic-dianhydride (Sigma-Aldrich, 284025) was added slowly while stirring and regulating to pH8. The solution was stirred for 2 h at 4 °C and was extensively dialyzed against 0.1 M sodium hydrogencarbonate using a ZelluTrans dialysis membrane (Carl Roth, E671.1). The obtained poly- L -lysine-DTPA was biotinylated by addition of 3 μmol EZ-Link NHS-Biotin. After 2 h of stirring at 4 °C the solution was dialyzed against 1 M citrate buffer (pH6.5). Six hundred micromol gadolinium chloride hexahydrate (Sigma-Aldrich, G7532) was dissolved in 0.1 M sodium acetate (pH6) and slowly added to the biotin-poly- L -lysine-DTPA solution. After 20 h of stirring at 4 °C, the solution was first dialyzed against 1 M citrate buffer (pH6.5) to remove free Gd 3+ ions within the solution followed by a dialysis against 0.1 M sodium hydrogencarbonat buffer. Then, 1 mg Alexa532 carboxylicacid-succinimidylester (Invitrogen, A-2010) was dissolved in 200 μl of dimethylsulphoxide and slowly added to the biotin-poly- L -lysine-Gd 3+ -DTPA solution. After stirring at 4 °C for 30 min, the free dye was removed while simultaneously concentrating the labelled probe using a Centriprep Ultracel (Millipore, YM.10). T 1 -decay fitting Recorded T 1 curves were fit with a bi-exponential function , as the decay exhibited two components with T 1,short << T 1,long and A long > A short . We attribute the shorter component ( T 1,short <15 μs) to a few clustered and thus very proximal NV pairs subjected to cross-relaxation. The relaxation rates Γ 1 and the corresponding relaxation times T 1 given in the text are determined by the main decay of the second and significantly longer T 1 component. How to cite this article: Steinert, S. et al. Magnetic spin imaging under ambient conditions with sub-cellular resolution. Nat. Commun. 4:1607 doi: 10.1038/ncomms2588 (2013).